Genome-wide profiles of CtBP link metabolism with genome stability and epithelial reprogramming in breast cancer The C-terminal binding protein (CtBP) is a NADH-dependent transcriptional repressor that links carbohydrate metabolism to epigenetic regulation by recruiting diverse histone-modifying complexes to chromatin. Here global profiling of CtBP in breast cancer cells reveals that it drives epithelial-to-mesenchymal transition, stem cell pathways and genome instability. CtBP expression induces mesenchymal and stem cell-like features, whereas CtBP depletion or caloric restriction reverses gene repression and increases DNA repair. Multiple members of the CtBP-targeted gene network are selectively downregulated in aggressive breast cancer subtypes. Differential expression of CtBP-targeted genes predicts poor clinical outcome in breast cancer patients, and elevated levels of CtBP in patient tumours predict shorter median survival. Finally, both CtBP promoter targeting and gene repression can be reversed by small molecule inhibition. These findings define broad roles for CtBP in breast cancer biology and suggest novel chromatin-based strategies for pharmacologic and metabolic intervention in cancer. Cancer evolves through a multi-step process driven by a global reprogramming of cellular gene expression patterns that confers adaptive advantages for tumour growth, proliferation and dissemination [1] . This phenotypic transformation is accomplished by diverse molecular strategies that control programs of cellular function by directing large-scale changes in gene expression [2] . Although our understanding of how specific genetic mutations can act as drivers of cancer is well established, the paradigms addressing how epigenetic changes are orchestrated to influence hallmarks of cellular malignancy are only just beginning to evolve [3] . Epigenetic changes represent potentially reversible covalent modifications to chromatin that can be transmitted to subsequent generations in the absence of changes to genetic sequence. In combination with DNA methylation and histone modifications (including acetylation, methylation, phosphorylation and ubiquitylation), these covalent modifications constitute a ‘histone code’ that is sculpted and interpreted by an assortment of chromatin regulatory complexes that bind (‘read’), place (‘write’) and remove (‘erase’) chromatin marks to create the living ‘libretto’ that we now refer to as the ‘epigenome’ [3] . How the spatial and kinetic distribution of these chromatin regulatory complexes are coordinated to influence the epigenome has become the focus of extensive investigation [4] . The C-terminal binding proteins (CtBP1/2) are a dimeric family of proteins encoded by two paralogous genes, CtBP1 and CtBP2 , that have extensive roles in animal cell development [5] . CtBP homo- and heterodimerize in the presence of NADH to recruit various chromatin-modifying complexes, including histone methyltransferases (HMTs), histone demethylases (HDMs) and histone deacetylases (HDACs) (for example, LSD1, HDAC1/2/4/6/7, G9a and EHMT) to chromatin-bound sequence-specific transcription factors [5] . In this way, CtBP has the potential to link metabolic status to specific changes in the epigenetic landscape of the nucleus and have a dominant role in determining cellular behaviour and fate [6] , [7] . However, with the exception of a small set of tumour suppressor genes (for example, CDH1 ( E-Cadherin ), CDKN2A ( p16 ), Sirtuin 1 and BRCA1 ) [6] , [8] , the genome-wide targets of CtBP in the mammalian nucleus remain unknown. Previously, we showed that CtBP repressed the transcriptional expression of the early-onset breast cancer gene, BRCA1, by recruiting HDAC activity to the BRCA1 promoter to antagonize p300-driven histone acetylation [8] . In this current work we extend this observation by profiling the global association of CtBP with the genome of breast cancer cells by combining chromatin immunoprecipitation with deep sequencing (ChIP-Seq) to define cellular programs driven by CtBP with clinical importance, and potential for therapeutic targeting. Here we reveal that CtBP has a prominent role in epigenetic reprogramming that drives major hallmarks of cancer through transcriptional mechanisms that are both linked to metabolism and susceptible to pharmacologic intervention. CtBP targets cellular reprograming and genome stability Recent molecular and morphological studies have shown that most breast cancers can be separated into distinct subtypes that segregate along the hierarchy of normal mammary epithelial differentiation and development, and include luminal A, luminal B, human epithelial growth factor receptor 2 (HER2) positive, basal-like and claudin low [9] , [10] . Luminal A and B are well-differentiated tumours and usually oestrogen receptor positive. The basal-like and claudin low subtypes are much more primitive and usually deficient in receptors for oestrogen and progesterone and HER2 (refs 9 , 10 ). This classification has substantial diagnostic and prognostic importance. The more primitive tumours (for example, basal-like and claudin low) usually show a more aggressive behaviour with worse clinical outcome [9] , [10] . Properties of these tumours include mesenchymal features associated with reactivation of embryonic programs that promote EMT, acquisition of stem cell-like self-renewal attributes, increased genome instability, and the production of cellular progenitors with the ability to seed new tumours, often referred to as ‘tumour-initiating cells’ (TICs) [11] , [12] , [13] . Such features are recognized as important hallmarks or drivers of cancer [1] . We profiled the binding of CtBP across the genome of the human breast cancer cell line MCF-7, a well-differentiated oestrogen receptor positive luminal subtype, using antibodies that recognize epitopes common to both CtBP1 and CtBP2 ( Fig. 1 ). Genome-wide ChIP-seq analysis identified a total of 6,607 binding sites for CtBP with a false discovery rate (FDR)<0.00001. 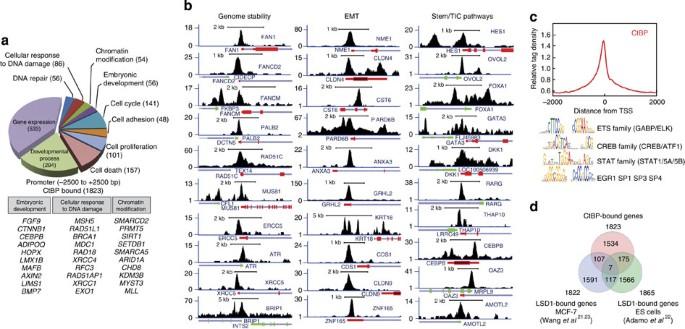Figure 1: Global targeting of genome stability and developmental pathways by CtBP differentiation. (a) Gene ontology analysis indicates that CtBP targets numerous cancer-related pathways linked to DNA repair, chromatin modifications, cell adhesion and other pathways important in developmental processes. (b) ChIP-Seq profiles of the binding of CtBP to selected genes that are key genetic drivers of human malignancy including genome stability, epithelial-to-mesenchymal transition (EMT) and stem cell/tumour initiation cell (TIC) pathways in MCF-7 cells. Red indicates genes encoded 5′–3′ on the upper strand, whereas green indicates genes encoded 5′–3′ on the lower strand. (c) Binding motifs enriched under CtBP ChIP-seq peaks revealed byin silicoanalysis. (d) The large majority of promoter binding sites for CtBP are distinct from those bound by LSD1 in MCF-7 and human ES cells. A total of 1,823 of these binding sites were in promoter regions ( Table 1 ). Consistent with the established role for CtBP in animal cell development [14] , ontology analysis of the 1,823 gene promoters demonstrates that CtBP interacts with gene networks that have broad roles in cellular homeostasis including cellular macromolecule metabolic processes, RNA processing, gene expression and cellular metabolic processes ( Supplementary Table S1 ). However, a large number of CtBP-targeted genes belong to categories that are important in malignant tumour transformation and progression, including embryonic development, cellular response to DNA damage, cell cycle, cell proliferation, cell death, cell adhesion and chromatin modifications ( Fig. 1a ). CtBP binding sites located outside of promoter regions are also nearby genes that show a similar distribution of these categories ( Supplementary Figs S1a–d ). In particular, many of the CtBP target genes belong to functional gene categories that have major roles in driving the more aggressive mesenchymal phenotypes of basal-like and claudin low tumours including genome instability, EMT and stem cell-like/TIC pathways [10] , [13] ( Fig. 1b ). The core list of 30 CtBP bound genes in Fig. 1b (10 from each category, each with Z -scores>30.17), include multiple genes that have been previously shown to have major roles in breast cancer aetiology, genetic susceptibility and tumour progression [15] , [16] . It was therefore selected for use in subsequent validation studies. Figure 1: Global targeting of genome stability and developmental pathways by CtBP differentiation. ( a ) Gene ontology analysis indicates that CtBP targets numerous cancer-related pathways linked to DNA repair, chromatin modifications, cell adhesion and other pathways important in developmental processes. ( b ) ChIP-Seq profiles of the binding of CtBP to selected genes that are key genetic drivers of human malignancy including genome stability, epithelial-to-mesenchymal transition (EMT) and stem cell/tumour initiation cell (TIC) pathways in MCF-7 cells. Red indicates genes encoded 5′–3′ on the upper strand, whereas green indicates genes encoded 5′–3′ on the lower strand. ( c ) Binding motifs enriched under CtBP ChIP-seq peaks revealed by in silico analysis. ( d ) The large majority of promoter binding sites for CtBP are distinct from those bound by LSD1 in MCF-7 and human ES cells. Full size image Table 1 Genome-wide binding sites for CtBP. Full size table In silico analysis of consensus binding motifs centred under CtBP peaks shows a large enrichment of transcription factor binding sites for ETS, CREB, STAT and EGR1/SP1 families of transcription factors ( Fig. 1c and Supplementary Fig. S2 ). Notably, these motifs are overrepresented in the promoters of both bidirectional and DNA repair genes including BRCA1, PALB2, FANCD2, FANCM and RAD51C [17] , [18] (also see Fig. 1b ). In addition, the ETS pathway has been identified as a major programme in basal-like breast cancers [19] . This finding suggests that CtBP recruitment is likely to be coordinated through a common promoter context to control specific cellular programs. CtBP is often found in complexes with the HDM, LSD1, where it has a broad role in both repressive and activating transcriptional programs in various cell types [20] , [21] , [22] . In breast epithelia, LSD1 represses invasion and metastasis [23] . However, comparison of the targets of CtBP and LSD1 in MCF-7 and human ES cells reveals less than a 7% and 10% overlap, respectively ( Fig. 1d ). This indicates that the major functions of CtBP in epigenetic regulation are likely to involve complexes that are distinct from LSD1 targeting in mammary epithelial cells. CtBP promotes EMT and enhances TIC traits Though CtBP predominantly produces repression of target genes, both the dimeric state of CtBP and composition of the CtBP-containing complex are major determinants of whether CtBP will repress or induce gene expression [21] , [24] , [25] . An analysis of the relative enrichment of CtBP-targeted genes in molecular signatures of EMT [26] shows a significant ( P =9.5 E-11) overlap with genes that are differentially repressed (downregulated) compared with activated (upregulated) during EMT ( Fig. 2a ). Similarly, CtBP-bound genes are significantly more enriched ( P =7.37E-10) in the genes that are differentially repressed in the cancer TIC/Stem cell signature [12] ( Fig. 2a ). These findings implicate a predominant role for CtBP in driving both EMT and stem cell-like attributes through transcriptional repression. 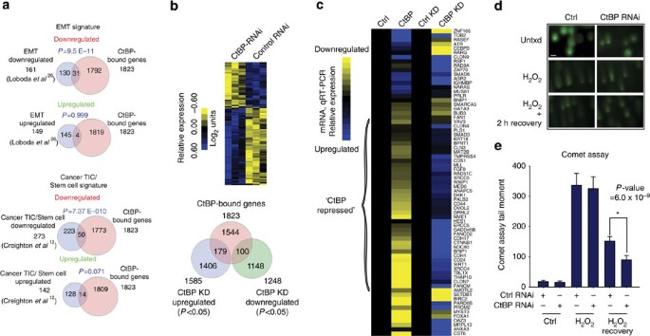Figure 2: CtBP downregulated targets control differentiation and DNA repair. (a) Venn diagrams showing the overlap between CtBP targets and genes downregulated and upregulated in established EMT and cancer tumour-initiating cell (TIC)/stem cell gene signatures.P-values indicate the significance of overlap determined from hypergeometric distribution analysis. (b) Unsupervised hierarchical clustering of microarray analysis (HGU133plus) of differentially expressed (P<0.05) genes in control and MCF-7 cells depleted of CtBP by RNAi. Venn diagram shows the overlap of repressed and induced genes with CtBP targets identified by ChIP-Seq. (c) Hierarchical clustering of the expression of multiple CtBP targets belonging to the gene classes, described inFig. 1, measured by quantitative real-time PCR in cells overexpressing CtBP (CtBP) and cells depleted of CtBP by RNAi (CtBP KD) compared with GFP control and non-targeting RNAi, respectively. Bracket indicates CtBP repressed genes that were uniformly upregulated by CtBP depletion and repressed by CtBP overexpression. Corresponding expression values with error bars are provided inSupplementary Figs S4–S6(d) Comet assay of MCF-7 cells before and after oxidative DNA damage by peroxide treatment and following 2 h recovery in control cells and cells depleted of CtBP by RNAi. (e) Analysis of change in tail moment in control and CtBP-depleted cells following DNA damage and recovery. The error bars represent the s.d. of the mean from two independent experiments. Scale bar, 20 μm. Figure 2: CtBP downregulated targets control differentiation and DNA repair. ( a ) Venn diagrams showing the overlap between CtBP targets and genes downregulated and upregulated in established EMT and cancer tumour-initiating cell (TIC)/stem cell gene signatures. P -values indicate the significance of overlap determined from hypergeometric distribution analysis. ( b ) Unsupervised hierarchical clustering of microarray analysis (HGU133plus) of differentially expressed ( P <0.05) genes in control and MCF-7 cells depleted of CtBP by RNAi. Venn diagram shows the overlap of repressed and induced genes with CtBP targets identified by ChIP-Seq. ( c ) Hierarchical clustering of the expression of multiple CtBP targets belonging to the gene classes, described in Fig. 1 , measured by quantitative real-time PCR in cells overexpressing CtBP (CtBP) and cells depleted of CtBP by RNAi (CtBP KD) compared with GFP control and non-targeting RNAi, respectively. Bracket indicates CtBP repressed genes that were uniformly upregulated by CtBP depletion and repressed by CtBP overexpression. Corresponding expression values with error bars are provided in Supplementary Figs S4–S6 ( d ) Comet assay of MCF-7 cells before and after oxidative DNA damage by peroxide treatment and following 2 h recovery in control cells and cells depleted of CtBP by RNAi. ( e ) Analysis of change in tail moment in control and CtBP-depleted cells following DNA damage and recovery. The error bars represent the s.d. of the mean from two independent experiments. Scale bar, 20 μm. Full size image To obtain a general impression of the correlation between CtBP promoter occupancy and gene expression, microarray analysis was used to compare gene expression patterns in control versus MCF-7 cells that had been depleted of CtBP by RNAi ( Fig. 2b ). This screen identified 1,585 genes that showed significant ( P <0.05) upregulation and 1,248 genes that showed downregulation by either direct or indirect CtBP influence. Using the FDR cutoff described above, 179 of the upregulated and 100 of the downregulated genes were identified as CtBP targets by ChIP-Seq. Although the specific functional distribution of differentially expressed gene classes is similar to the ChIP-Seq distribution shown in Fig. 1a ( Supplementary Fig. S7 ), the modest size of the overlap is likely a reflection of direct and indirect influences of CtBP depletion in combination with the insensitivity and low dynamic range of hybridization-based array technology [27] . Therefore, to generate a more accurate view of the relationship between CtBP occupancy and gene expression, a total of 71 genes (30 genes from Fig. 1b and 41 additional genes collected from gene categories described in Fig. 1 ; in total representing 26% of the EMT overlap and 38% of the TIC overlap in Fig. 2a ) were selected for validation by quantitative mRNA expression (quantitative reverse transcription–PCR) and quantitative ChIP. Both cells depleted of CtBP by RNAi and cells overexpressing CtBP were analysed and compared ( Fig. 2c and Supplementary Figs S3–S6 ). By this analysis, 56% of the validation genes showed significant ( P <0.05) upregulation following CtBP depletion, whereas 14% showed downregulation ( Supplementary Figs S4–S6 ). Conversely, 46% of genes in cells overexpressing CtBP showed significant repression ( P <0.05), whereas 15% showed upregulation. Hundred percentage of genes tested by quantitative ChIP showed a significant peak ( P <0.05) and 90% (27 of 30) genes showed a significant decrease ( P <0.05) of CtBP binding following CtBP gene depletion by RNAi ( Supplementary Figs S3 and S6 ). These data show that many of the genes identified by ChIP-Seq analysis are likely to be bona fide functional targets of CtBP. Global depletion of CtBP increases DNA repair CtBP-bound sequences are enriched in transcription factor binding sites found in the promoters of genes involved in DNA repair ( Fig. 1b ). Many of these are derepressed following CtBP depletion ( Fig. 2c and Supplementary Fig. S4 ). These findings, in combination with the previously reported repressive effects of CtBP on BRCA1 expression [8] , suggests that CtBP levels may have a strong influence on DNA repair. To test this, comet assays were performed on MCF-7 cells exposed to oxidative DNA damage before or after CtBP gene depletion by RNAi ( Fig. 2d ). Analysis reveals that cells depleted of CtBP show significantly increased DNA repair ( P =6.0 E-09) compared with control cells ( Fig. 2e ). In contrast, gene depletion of BRCA1 by RNAi has the opposite effect (decreased DNA repair), though with lower relative significance ( P =1.50 E-05) ( Supplementary Fig. S8 ). These findings establish a substantial role for CtBP in governing transcriptional programs that control genome stability. CtBP drives acquisition of mesenchymal traits To assess the functional influence of CtBP on the acquisition of mesenchymal traits, we compared the effect of CtBP expression on the properties of two cell lines at opposite poles of the hierarchy of mammary differentiation ( Fig. 3 ). MCF-7 cells serve as a representative of luminal differentiation, whereas MDA-MB-231, an oestrogen receptor negative and highly metastatic cell line, is representative of the claudin low subtype. In both cell lines, CtBP depletion induces derepression of most of the 30 CtBP-targeted genes in Fig. 1b ; however, gene depletion seems to derepress a substantially larger portion of the MDA-MB-231 cells than the MCF-7 (80% versus 53%) ( Fig. 3a and Supplementary Fig. S4 ). In contrast, CtBP overexpression has a more substantial influence on the repression of the 30 CtBP targets in MCF-7 compared with MDA-MB-231 (43% versus 6%) ( Fig. 3a and Supplementary Fig. S5 ). CtBP is associated with a variety of chromatin-modifying complexes [5] . At the BRCA1 promoter, loss of CtBP results in increased BRCA1 promoter acetylation and increased BRCA1 expression [8] . However, in the absence of direct empirical information or further study of the specific forms of CtBP complexes in different cell types or knowledge of the differential promoter recruitment of histone acetyl-transferase, HDACs, HMTs and HDMs, it is not possible to readily predict what modifications will be altered and in what direction at each individual CtBP target. Regardless, CtBP gene depletion produces substantial changes in both H3 and H4 histone acetylation at most of the 30 CtBP gene targets ( Fig. 3c and Supplementary Fig. S9 ). 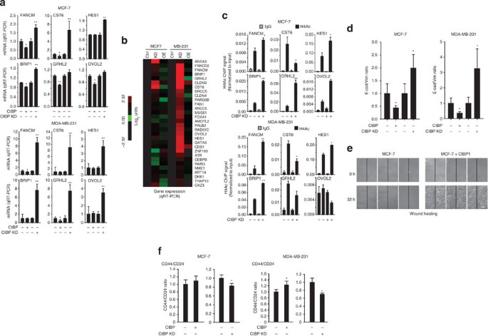Figure 3: CtBP drives acquisition of mesenchymal traits in mammary epithelial cells. (a) Gene expression pattern of CtBP target genes controlling genome stability, EMT and stem cell pathways in MCF-7 cells (top) and MDA-MB-231 cells (bottom) overexpressing CtBP or depleted of CtBP by RNAi as indicated. (b) Unsupervised hierarchical clustering comparing of the 30 gene validation set expression (seeFig. 1b) in cells overexpressing or depleted of CtBP. Expression values with error bars are shown inSupplementary Figs S4,S5. (c) Promoter Histone H4 acetylation profile (K5, K8, K12, K16) of genes shown inain MCF-7 cells (top) and MDA-MB-231 cells (bottom) following CtBP depletion by RNAi. Expression values and errors bars including the remaining 30 gene validation set are provided inSupplementary Fig. S9. (d) E-cadherin/Vimentin expression ratio in cells overexpressing CtBP or depleted of CtBP by RNAi. (e) Wound-healing assay shows MCF-7 control cells and cells overexpressing CtBP1. Vertical line indicates centre of wound in the scratch assay. White bar, 250 μm. (f) CD44/CD24 expression ratio in MCF-7 and MDA-MB-231 cells overexpressing CtBP or depleted of CtBP by RNAi. The error bars represent the s.d. of the mean from three independent experiments (a,d,f) or two independent experiments (c). *indicatesP<0.05 and **indicatesP<0.01. Figure 3: CtBP drives acquisition of mesenchymal traits in mammary epithelial cells. ( a ) Gene expression pattern of CtBP target genes controlling genome stability, EMT and stem cell pathways in MCF-7 cells (top) and MDA-MB-231 cells (bottom) overexpressing CtBP or depleted of CtBP by RNAi as indicated. ( b ) Unsupervised hierarchical clustering comparing of the 30 gene validation set expression (see Fig. 1b ) in cells overexpressing or depleted of CtBP. Expression values with error bars are shown in Supplementary Figs S4,S5 . ( c ) Promoter Histone H4 acetylation profile (K5, K8, K12, K16) of genes shown in a in MCF-7 cells (top) and MDA-MB-231 cells (bottom) following CtBP depletion by RNAi. Expression values and errors bars including the remaining 30 gene validation set are provided in Supplementary Fig. S9 . ( d ) E-cadherin/Vimentin expression ratio in cells overexpressing CtBP or depleted of CtBP by RNAi. ( e ) Wound-healing assay shows MCF-7 control cells and cells overexpressing CtBP1. Vertical line indicates centre of wound in the scratch assay. White bar, 250 μm. ( f ) CD44/CD24 expression ratio in MCF-7 and MDA-MB-231 cells overexpressing CtBP or depleted of CtBP by RNAi. The error bars represent the s.d. of the mean from three independent experiments ( a , d , f ) or two independent experiments ( c ). *indicates P <0.05 and **indicates P <0.01. Full size image A well-characterized attribute of the acquisition of mesenchymal features and EMT is increasing vimentin expression accompanied by decreasing E-cadherin expression [11] . To profile the influence of CtBP on these properties, the change in the E-cadherin/Vimentin ratio [28] was measured ( Fig. 3d ). In both MCF-7 cells and MDA-MB-231 cells, CtBP gene depletion increased the ratio of E-cadherin/Vimentin, whereas CtBP expression lowered it, consistent with the ability of CtBP to drive the mesenchymal phenotype in both mesenchymal and luminal cells. Furthermore, the role of CtBP in driving mesenchymal features is well illustrated by the ability of enforced CtBP expression to substantially increase MCF-7 mobility in wound-healing assays ( Fig. 3e ). EMT has recently been shown to activate programs that promote the acquisition of stem cell-like properties [11] . This often occurs in progenitor cells with increases in CD44 as opposed to CD24 expression [11] . The influence of CtBP on stem-like features of MCF-7 and MDA-MB-231 was measured by profiling changes in the CD44/CD24 ratio [10] following enforced CtBP expression or CtBP gene depletion ( Fig. 3f ). In both cell lines, the expression of CtBP increased the CD44/CD24 ratio consistent with the attributes of cells with progenitor/stem cell-like features, whereas CtBP depletion decreased that ratio ( Fig. 3f ). Thus, CtBP appears to be able to drive the mesenchymal phenotype in mammary cells regardless of what position they are along the spectrum of mammary differentiation. CtBP links cellular metabolic status to genome stability Pharmacological manipulation of endogenous NADH levels influences BRCA1 expression through CtBP, with higher levels of NADH causing BRCA1 repression [8] . To ask whether manipulation of endogenous NADH levels by carbohydrate over-loading could influence expression of CtBP targets, we grew MCF-7 cells in high or ‘diabetic’ levels of glucose (450 mg dl −1 ) versus normal concentration (100 mg dl −1 ) ( Fig. 4 ). CtBP dimerization, nuclear localization, and stability are enhanced when bound to NADH [7] , [29] . As demonstrated by both immunohistochemistry and western blot analysis, MCF-7 cells grown in low levels of glucose, demonstrate decreased levels of NADH relative to NAD+, and show lower nuclear accumulation of CtBP in comparison with cells grown under conditions of high glucose ( Fig. 4a–c ). These changes are, in turn, associated with increased nuclear levels of BRCA1 protein, decreased levels of CtBP loading at the BRCA1 promoter, compensatory increases in relative histone 4 acetylation [8] ( Fig. 4c–e and Supplementary Fig. S10a ) and a significant increase in the expression of BRCA1 mRNA and other CtBP-targeted genes important in DNA repair ( Fig. 4f and Supplementary Fig. S10b ). Finally, as predicted, cells incubated under high glucose condition show a demonstrably reduced DNA repair capacity, which is not due to differences in cell cycle entry ( Fig. 4g and Supplementary Fig. S10c ). 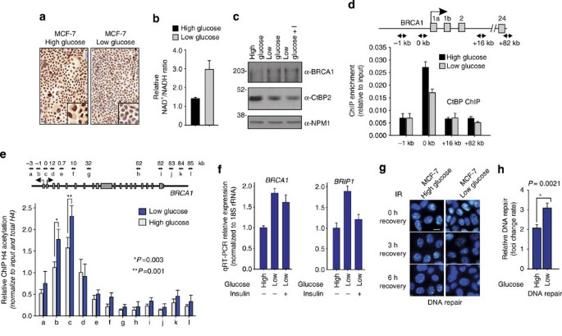Figure 4: Calorie restriction decreases CtBP activity and increases DNA repair. (a) CtBP immunohistochemical staining of MCF-7 cells grown in high glucose (4.5 g l−1) and low glucose (1.0 g l−1). Scale bar, 25 μm. Inset is two-fold magnification. (b) NAD+/NADH ratio in lysates of MCF-7 cells grown in high and low glucose. (c) Western blot analysis of BRCA1 and CtBP2 expression in high and low glucose-treated cells. NPM1 was used as loading control. I, insulin. (d) ChIP profile of CtBP binding to the BRCA1 promoter in cells grown in high glucose versus low glucose as indicated. (e) ChIP profile of relative histone 4 lysine acetylation after normalization to ChIP for total histone 4. (f) Quantitative reverse transcription–PCR expression ofBRCA1andBRIP1mRNA in high and low glucose-treated cells with and without insulin. (g) Phospho-gamma H2AX foci profile of cells following ionizing radiation at 0, 3 and 6 h. Scale bar, 10 μm. (h) Relative rate of DNA repair expressed as relative rate of decrease in foci per cell over time. The error bars represent the s.d. of the mean from three independent experiments (b,d,f,h) or five independent experiments (e). Figure 4: Calorie restriction decreases CtBP activity and increases DNA repair. ( a ) CtBP immunohistochemical staining of MCF-7 cells grown in high glucose (4.5 g l −1 ) and low glucose (1.0 g l −1 ). Scale bar, 25 μm. Inset is two-fold magnification. ( b ) NAD + /NADH ratio in lysates of MCF-7 cells grown in high and low glucose. ( c ) Western blot analysis of BRCA1 and CtBP2 expression in high and low glucose-treated cells. NPM1 was used as loading control. I, insulin. ( d ) ChIP profile of CtBP binding to the BRCA1 promoter in cells grown in high glucose versus low glucose as indicated. ( e ) ChIP profile of relative histone 4 lysine acetylation after normalization to ChIP for total histone 4. ( f ) Quantitative reverse transcription–PCR expression of BRCA1 and BRIP1 mRNA in high and low glucose-treated cells with and without insulin. ( g ) Phospho-gamma H2AX foci profile of cells following ionizing radiation at 0, 3 and 6 h. Scale bar, 10 μm. ( h ) Relative rate of DNA repair expressed as relative rate of decrease in foci per cell over time. The error bars represent the s.d. of the mean from three independent experiments ( b , d , f,h ) or five independent experiments ( e ). Full size image CtBP gene networks distinguish aggressive breast cancer The embryonic properties linked to EMT, including cellular plasticity, dedifferentiation, deregulated cell growth and genome instability, are common features associated with more aggressive molecular subtypes of breast cancer [30] , [31] . To ask whether CtBP target genes define networks that are more associated with aggressive subtypes of breast cancer, we profiled the expression of CtBP target genes in publically available breast cancer patient gene expression data sets ( Fig. 5a ). Analysis by unsupervised hierarchical clustering identified a large class or cluster of CtBP-targeted genes that are selectively downregulated in the basal-like and claudin low subtype of cancers ( Fig. 5a ). Moreover, ANOVA (analysis of variance) analysis [10] of expression of the CtBP-targeted gene categories ( Fig. 1b ), shows that downregulation of many of the genes within the EMT and Stem Cell/TIC categories significantly distinguish ( P -values between 1.08 E-11 and 1.17 E-140) basal-like and claudin low from the other subtypes ( Fig. 5b and Supplementary Fig. S11 ). GRHL2 has recently been shown to have a dominant role in EMT by regulating cell polarity and is a strong discriminator of claudin low subtypes [32] , [33] . FOXA1 potently distinguishes basal-like and claudin low from the more luminal subtypes and has recently been shown to actively repress the basal-like phenotype [34] , [35] ( Figs 1b and 5b and Supplementary Fig. S11 ). Similarly, gene set enrichment analysis [36] of the genes altered by CtBP RNAi depletion using microarray analysis ( Fig. 2b ) also reveals substantial CtBP-dependent participation in multiple pathways important in breast cancer biology ( Supplementary Figs S12a–g ) [37] . Moreover, the clinical relevance of the CtBP-targeted gene list is further supported by analysis of two independent breast cancer gene expression studies revealing that patients, whose tumours can be classified as showing differential expression of CtBP-target genes, have significantly shorter metastasis-free survival by Kaplan–Meier analysis ( Fig. 5c ). 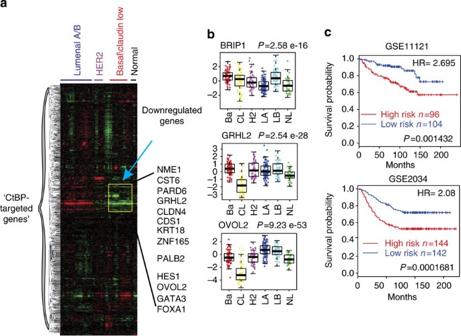Figure 5: CtBP targets distinguish clinically aggressive subtypes of breast cancer. (a) Unsupervised hierarchical clustering of CtBP target genes in publically available breast cancer gene expression studies (UNC337). Highlighted rectangle indicates group of CtBP-bound genes that are downregulated/repressed preferentially in the basal-like subtype. (b) ANOVA profiling of one representative each of the genome stability (BRIP1), EMT (GRHL2) and TIC/Stem cell (OVOL2) gene groups, described inFig. 1b, using the UNC337 patient gene expression data set.P-values were calculated by comparing mean expression across all subtypes. (c) Patients whose tumours differentially express CtBP-bound genes show worse clinical outcome (metastasis-free survival) by Kaplan–Meier analysis. Patient gene expression data obtained from the Gene Expression Omnibus (GSE11121 and GSE2034) were separated into two groups based on differential expression CtBP target genes (red), and were analysed by Kaplan–Meier analysis. The 95% confidence interval for median hazard ratio (HR)=2.08 is (1.420, 3.070). The 95% confidence interval for median HR=2.70 is (1.490, 5.411).P-values and HRs were derived as described in Methods. Figure 5: CtBP targets distinguish clinically aggressive subtypes of breast cancer. ( a ) Unsupervised hierarchical clustering of CtBP target genes in publically available breast cancer gene expression studies (UNC337). Highlighted rectangle indicates group of CtBP-bound genes that are downregulated/repressed preferentially in the basal-like subtype. ( b ) ANOVA profiling of one representative each of the genome stability ( BRIP1 ), EMT ( GRHL2 ) and TIC/Stem cell ( OVOL2 ) gene groups, described in Fig. 1b , using the UNC337 patient gene expression data set. P -values were calculated by comparing mean expression across all subtypes. ( c ) Patients whose tumours differentially express CtBP-bound genes show worse clinical outcome (metastasis-free survival) by Kaplan–Meier analysis. Patient gene expression data obtained from the Gene Expression Omnibus (GSE11121 and GSE2034) were separated into two groups based on differential expression CtBP target genes (red), and were analysed by Kaplan–Meier analysis. The 95% confidence interval for median hazard ratio (HR)=2.08 is (1.420, 3.070). The 95% confidence interval for median HR=2.70 is (1.490, 5.411). P -values and HRs were derived as described in Methods. Full size image High CtBP predicts poor survival in breast cancer patients The data presented thus far indicate that CtBP is likely to have a substantial role in the aetiology and progression of human breast cancer. To examine CtBP expression in patient tissues, tumour samples from breast cancer patients were stained for CtBP protein expression by immunohistochemistry using antibodies against CtBP ( Fig. 6a ). In normal breast CtBP, nuclear immunoreactivity is generally light and non-uniform with many nuclei showing little or no CtBP staining, whereas in patients with basal-like, triple-negative breast cancer, CtBP1 staining is much more intense ( Fig. 6a ). When digitally scored for CtBP nuclear staining to measure percent of nuclei with scores of 0–3 (nuclear intensity) or a score weighted by nuclear size (nuclear score), triple-negative breast cancer shows a nuclear intensity and nuclear score that is 25 and 22 times higher than normal breast, respectively ( Fig. 6a ). This system was then used to score the patient tissue cohort ( Fig. 6b ). When this scoring system was used to segregate patient samples into three groups of low (nuclear score <100; nuclear intensity <2), medium (nuclear score 100–300; nuclear intensity 2–5) and high (nuclear score >300; nuclear intensity >5) CtBP score, there was a clear trend showing an inverse relationship between CtBP staining and patient median survival by Kaplan–Meier analysis ( Fig. 6b ). This suggests that elevated CtBP has potential as a surrogate biomarker for altered epigenetic regulation in breast cancer patients who may progress to more advanced disease, although the prognostic value of CtBP will require further independent validation. 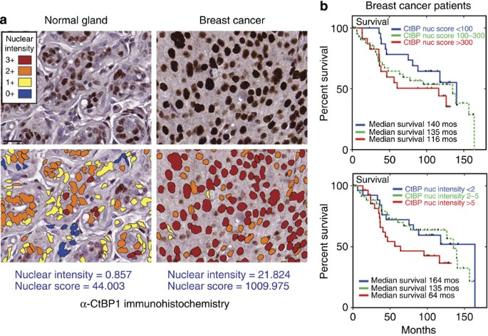Figure 6: Elevated CtBP protein in patient breast cancers predicts lower median survival. (a) CtBP1 immunohistochemical staining of normal breast tissue and tissue from triple-negative breast cancer patients, analysed for staining intensity using the Aperio nuclear algorithm software and then scored for nuclear intensity and nuclear score (weighted by nuclear area). Scale bar, 25 μm. (b) Relative survival of a breast cancer patient cohort (98) scored with low (<100 or <2.0), median (100–300 or 2–5) and high (>300 or>5) scores for CtBP staining analysed for survival trends by Kaplan–Meier analysis. Median survival for all three groups are shown. Cox regression analysis of hazard ratio for nuclear intensity >5 is 2.10 (P-value=0.048) after adjusting for age. Figure 6: Elevated CtBP protein in patient breast cancers predicts lower median survival. ( a ) CtBP1 immunohistochemical staining of normal breast tissue and tissue from triple-negative breast cancer patients, analysed for staining intensity using the Aperio nuclear algorithm software and then scored for nuclear intensity and nuclear score (weighted by nuclear area). Scale bar, 25 μm. ( b ) Relative survival of a breast cancer patient cohort (98) scored with low (<100 or <2.0), median (100–300 or 2–5) and high (>300 or>5) scores for CtBP staining analysed for survival trends by Kaplan–Meier analysis. Median survival for all three groups are shown. Cox regression analysis of hazard ratio for nuclear intensity >5 is 2.10 ( P -value=0.048) after adjusting for age. Full size image Reversal of CtBP function by small molecule inhibition CtBP is a potent epigenetic regulator that responds to cellular metabolism through its interaction with NADH. Therefore, pharmacological targeting of CtBP may, in principle, provide a means of derepressing its transcriptional targets. Though CtBP is a member of the d-2-hydroxyacid dehydrogenase family, its true substrate is not known [38] . Recent studies indicate that 2-Keto-4-methylthiobutyrate (MTOB), an intermediate in the methionine salvage pathway, can bind CtBP and reverse repression of the proapoptotic gene, BIK, in colon cancer cells [39] , [40] . To test whether MTOB could disrupt expression of CtBP target genes in breast cancer, both MCF-7 and MDA-MB-231 were incubated in the presence and absence of MTOB and the 30 CtBP-targeted genes ( Fig. 1b ) were screened for changes in gene expression ( Fig. 7a and Supplementary Fig. S13 ) and promoter occupancy ( Fig. 7d and Supplementary Figs S14,S15 ). MTOB treatment caused significant derepression ( P <0.05) of 40% of these genes in MCF-7 and 46% in MBA-MD-231. Approximately 3% and 10% of genes, respectively, were repressed ( Fig. 7a and Supplementary Fig. 13 ). The concordance of the MTOB effect between the two cell lines was 70% (21/30), indicating that MTOB action is relatively independent of breast cancer subtype and epithelial programming ( Fig. 7b and Supplementary Fig. S13 ). However, though it is difficult to know the extent to which this derepression is due to direct targeting of CtBP occupancy or to indirect effects; incubation with MTOB caused a significant displacement ( P <0.05) of CtBP from 67% of the promoters in MCF-7 and only 30% from promoters in MDA-MB-231 ( Fig. 7d and Supplementary Fig. S14 ). The lower MTOB-induced CtBP displacement in MDA-MB-231 could be due to the lower level of CtBP binding found at these genes ( Supplementary Fig. S3 ). This could explain, in part, why the concordance between changes in CtBP occupancy and gene expression is significantly higher for MCF-7 (>70%) compared with MDA-MB-231 (50%) following MTOB treatment ( Fig. 7a and Supplementary Figs S13–S15 ). Nonetheless, these data indicate that the predominant mode of MTOB action is through its eviction of CtBP from occupied promoter regions. Finally, treatment with MTOB antagonizes the mesenchymal phenotype ( Fig. 7e ). Addition of MTOB to both MCF-7 and MDA-MD-231 increases the pro-epithelial E-cadherin/Vimentin ratio while reducing the pro-mesenchymal CD44/CD24 ratio, with a more significant trend ( P <0.05) in MCF-7 ( Fig. 7e ). Taken all together, these findings provide substantial evidence that pharmacological targeting of CtBP to disrupt malignant cellular reprogramming may be a feasible ‘epigenetic strategy’ for therapeutic intervention. 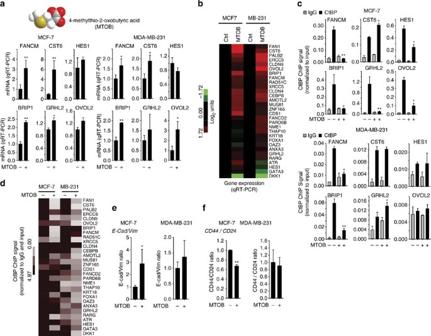Figure 7: Small molecule inhibition reverses gene repression by CtBP eviction. (a) Gene expression pattern of CtBP target genes controlling genome stability, EMT and stem cell pathways in MCF-7 cells (left) and MDA-MB-231 cells (right) with and without treatment with 10 mM MTOB. (b) Heat map of gene expression of the 30 gene validation set (Fig. 1b) in MCF-7 (left) and MDA-MB-231 (right) cells treated with and without MTOB. Gene expression values and error bars including the remaining 30 genes are provided inSupplementary Fig. S13. (c) CtBP qChIP profiles of genome stability, EMT and stem cell pathways genes in MCF-7 (top) and MDA-MB-231 (bottom) cells treated with or without MTOB. (d) Heat map of ChIP intensities of 30 gene validation list in MCF-7 and MDA-MB-231 cells treated with or without MTOB. Quantitative ChIP values and error bars are provided inSupplementary Fig. S14. (e) E-cadherin/Vimentin ratio in MCF-7 and MDA-MB-231 cells treated with and without MTOB. (f) CD44/CD24 ratio in MCF-7 and MDA-MB-231 cells treated with and without MTOB. The error bars represent the s.d. of the mean from three independent experiments (a,e,f) or two independent experiments (c). *IndicatesP<0.05 and **indicatesP<0.01. Figure 7: Small molecule inhibition reverses gene repression by CtBP eviction. ( a ) Gene expression pattern of CtBP target genes controlling genome stability, EMT and stem cell pathways in MCF-7 cells (left) and MDA-MB-231 cells (right) with and without treatment with 10 mM MTOB. ( b ) Heat map of gene expression of the 30 gene validation set ( Fig. 1b ) in MCF-7 (left) and MDA-MB-231 (right) cells treated with and without MTOB. Gene expression values and error bars including the remaining 30 genes are provided in Supplementary Fig. S13 . ( c ) CtBP qChIP profiles of genome stability, EMT and stem cell pathways genes in MCF-7 (top) and MDA-MB-231 (bottom) cells treated with or without MTOB. ( d ) Heat map of ChIP intensities of 30 gene validation list in MCF-7 and MDA-MB-231 cells treated with or without MTOB. Quantitative ChIP values and error bars are provided in Supplementary Fig. S14 . ( e ) E-cadherin/Vimentin ratio in MCF-7 and MDA-MB-231 cells treated with and without MTOB. ( f ) CD44/CD24 ratio in MCF-7 and MDA-MB-231 cells treated with and without MTOB. The error bars represent the s.d. of the mean from three independent experiments ( a , e , f ) or two independent experiments ( c ). *Indicates P <0.05 and **indicates P <0.01. Full size image The evidence of a link between obesity and diabetes and increased mortality from breast cancer is incontrovertible [41] , [42] , [43] , [44] . An important feature of the dysfunctional energetics associated with obesity and diabetes and malignant transformation, is elevated carbohydrate metabolism, a central component of the Warburg effect [45] , [46] . This elevated level of carbohydrate metabolism, whether due to the over-nutrition of obesity or the Warburg effect of cancer bioenergetics, results in increased levels of NADH [47] , [48] , [49] . In this study, we propose CtBP is a key downstream epigenetic effector of elevated NADH. Therefore through CtBP, changes in cellular metabolic status can drive genome-wide changes in chromatin through targeted recruitment of CtBP that facilitates the acquisition of epigenetically reprogrammed properties that promote genome instability, dedifferentiation and the transformation to a more mesenchymal phenotype. Though this study provides one of the first to profile the binding of CtBP throughout the mammalian genome, how, when and where the different CtBP complexes target and coordinate the recruitment of specific chromatin modifiers, and their subsequent effect on the epigenome remain to be defined. These epigenetic networks and programs are likely to differ by cellular process and cell type and are likely to reflect a hierarchy of CtBP complexes formed under specific cellular conditions and environments as we have seen in comparing the mesenchymal MDA-MB-231 cell line with the luminal MCF-7 ( Figs 3 and 7 ). This difference has been demonstrated in prior studies where loss of CtBP had a much great effect on mitotic fidelity in MDA-MB-231 than MCF-7 [50] . Future studies to correlate global alterations in histone and DNA modification with changes in CtBP levels (via either genetic or metabolic disruption) in multiple breast cancer subtypes will be necessary to better define the mechanism underlying these differences. Approximately 5–10% of breast cancers are secondary to inherited mutations of cancer predisposing genes. It is striking that, of the known and newly identified breast cancer predisposing genetic mutations, a substantial number are targeted for repression by CtBP, including PALB2 , BRIP1 , RAD51C and BRCA1 (ref. 16 ). Thus, the observation that many patients develop breast cancers with features of inherited disease without demonstrating mutation in genes characteristic of the disease [51] , is consistent with a role CtBP-regulated pathways had in such tumours. Notably, decreased expression specifically of DNA repair proteins is associated with shortened time to recurrence in triple-negative breast cancer [52] . This is consistent with the demonstration, in this current study, of the impact of CtBP targeting on genome stability. Nearly one third of the Fanconi Anaemia complementation group is targeted by CtBP. Therefore, it is not surprising that loss of CtBP expression or function results in a significant improvement in DNA repair in breast cancer cell lines (see Figs 1d and 2d ). Most importantly, targeting by CtBP suggests that these hereditary risk factors for breast cancer may be worsened by lifestyle factors influencing metabolic imbalance. Finally, many of the new driver mutations identified by recent systematic sequencing of cancer genomes has uncovered several genes with functional roles in epigenetic regulation [53] . CtBP represents a novel class of versatile, multi-potent epigenetic regulators that is likely to have many different roles in cancer aetiology and progression. The finding that MTOB can act as a small molecular inhibitor that can reverse genomic targeting by CtBP, provides a proof of principle that pharmacological manipulation of CtBP is feasible. Thus, epigenetic targeting through CtBP promises to be a new and exciting area of future therapeutic intervention. New efforts will have to be directed at finding compounds that will function in the nanomolar to micromolar range. Given that weight gain and obesity represent modifiable cancer risk factors linked to lifestyle, a better understanding of CtBP will fuel new ideas and creative strategies for combined behavioural and therapeutic approaches to cancer treatment and prevention. Reagents Hydrogen peroxide is from Invitrogen as 30% stock. MTOB (4-methylthio-2-oxobutyric Acid ) is from Sigma-Aldrich and was dissolved in medium to 250 mM and diluted to 10 mM final concentration in cell culture. The antibody to CtBP used for ChIP was purchased from Santa Cruz Biotechnology and is cross-reactive with both CtBP1 and CtBP2. The anti-CtBP1-specific antibody and anti-CtBP2 specific antibody were purchased from BD biosciences. Anti-acetylated histone H3, anti-acetylated histone H4 antibodies and anti-γH2AX antibody were obtained from Millipore. Cell culture and tissues Both MCF-7 cells and MDA-MB-231 cells were maintained in regular DMEM supplemented with 10% (v/v) FBS, penicillin–streptomycin (Invitrogen) and insulin. In addition, the regular DMEM has 4.5 g l −1 glucose and is considered as high glucose culturing (HG) compared with 1.0 g l −1 glucose DMEM medium (LG). The low glucose-cultured cells were used for experiments only after 3 months of continuous culture in low-glucose medium. ChIP and ChIP-seq All ChIP experiments were carried out as described [8] . The detailed procedure is provided in the Supplementary Methods . ChIP-seq data analysis The detailed ChIP-seq data analysis is provided in the Supplementary Methods . Briefly, the 36-mer short-read tags were mapped to the human genome (UCSC HG19). Enrichment of tags in a 250 bp target window relative to a 200 kb surrounding window (local background) was gauged by a model based on the binomial distribution. The hotspots are defined by a z -score calculated using the target window and the background window signals both centred on the tag. In addition, ChIP hotspots were refined into 150 bp peaks using a peak-finding procedure. The sequencing data from matching input samples are used for the processing of the ChIP data, as a measure of background signal. Motif discovery and enrichment analysis A motif discovery analysis was performed on selected DNA sequences using MEME [54] on parallel clusters at the NIH Biowulf supercomputing facility. DNA sequences for MEME input were from the top 1,500 (by tag density) hotspots among all CtBP binding hotspots. To limit the computational load, only the 200 bp regions with the highest tag density were used instead of the entire width of a hotspot in cases where the hotspot spanned >200 bp. The width of motifs to discover was set to 6 and 20 for minimum and maximum, respectively. To identify motifs for known transcription factor binding, individual position-specific probability matrices against the Transfac database were queried using the TomTom software ( http://meme.nbcr.net/meme/cgi-bin/tomtom.cgi ). Statistically significant matches were retrieved that share the majority of specific nucleotides in the sequence motifs. To generate consensus read densities for positions relative to transcription start sites (TSS), the total number rd* of read tags summed over all Refseq annotated TSS normalized to the length L of the genome and the total number N of aligned reads (rd*=rd*L/N) was profiled such that rd*=1 approximately corresponds to an un-enriched distribution of reads. Gene expression and microarray analysis The total RNA from three biological replicates of control MCF-7 cells and CtBP knockdown MCF-7 cells were prepared using the RNAeasy kit (Qiagen) following the manufacturer’s protocol. Synthesis of cDNA from total RNA and hybridization/scanning of microarrays were performed with Affymetrix GeneChip products (HGU133plus2) as described in the GeneChip manual. Raw data files (.CEL) were converted into probe set values by Robust Mult-array Average (RMA) normalization. Following RMA normalization, Bioconductor packages was applied in R statistical environment to generate a list of genes that are differentially expressed between control cells and CtBP knockdown cells and P <0.05 was considered as significant. The data was stored as NCBI GSE36529. Comet assay Comet assays were performed according to Olive et al. [55] Briefly, a single-cell suspension was prepared using enzyme disaggregation. The cells were exposed to neutral lysis buffer (2% sarkosyl, 0.5M Na 2 EDTA, 0.5 mg ml −1 proteinase K (pH 8.0); equilibrated at 4 °C) for overnight at 37 °C. Following electrophoresis the cells were stained by SYBR Green and the images were obtained using fluorescent microscopy. The tail moment was calculated by the following formula: Tail moment=tail length × percentage of Tail DNA. Percentage of Tail DNA=aT × iT/(aT × iT+aH × iH), where aT=the tail area, iT=average intensity of tail, aH=the head area and iH=average intensity of Head. Comet Score was used to analyse the comet pictures. Immunofluorescence staining of cells Cells were grown on coverslips and fixed in 3.5% paraformaldehyde. For γH2AX staining the cells were incubated with Alexa Fluor 488 Goat Anti-Mouse IgG for 1 h. Cells were irradiated at 10 Gy to induce DNA damage. Immunohistochemistry staining of tissues Detailed methods for immunohistochemistry is provided in the Supplementary Methods . Formalin-fixed, paraffin-embedded tissues were de-paraffinized by submerging the slides in xylene. Antigen retrieval was performed in buffers containing 100 ml of 1 mM EDTA (pH 8.0). Staining was developed using secondary antibody conjugated with horse-radish peroxidase (HRP) (Dako EnVision)+System-HRP Labelled Polymer Anti-Rabbit or Anti-mouse and counterstained with haematoxylin. Analysis of tissue microarrays Immunohistochemically stained tissue slides were converted to digital slide images by scanning the slides on an Aperio ScanScope XT slide scanner. High-resolution digital slide images were then archived into Aperio’s digital pathology information management system ‘Spectrum’. Digital slide images were analysed using Aperio’s IHC Nuclear Image Analysis algorithm to assess the nuclear staining for CtBP in MCF7 cells and quantify the intensity of individual cells. Values and colours are assigned to individual cells based on the intensity of nuclear staining with a classification of 0 (blue), 1+ (yellow), 2+ (orange) and 3+ (red). Nuclear intensity was calculated from the sum of the product of the % of cells with 3+ and 2+ scores divided by the sum of the product of % cells with 1+ and 0 scores. Nuclear score was calculated as the product of nuclear area (μm 2 ) and the nuclear intensity. Archival formalin-fixed, paraffin-embedded tissues from breast cancer patients were obtained from the surgical pathology archive of the University of Chicago for tissue microarray construction. The study was approved by the Institutional Review Board of the University of Chicago and East Carolina University. Pathological features, including histological diagnosis, grade, tumour size and axillary lymph node metastasis, were abstracted from the pathology report. There were survival data on 98–100 breast cancer patients from each data set with a median follow-up of 8.3 years. Analysis of breast cancer gene expression profiles Expression patterns of the 1,823 genes identified by CtBP ChIP-Seq were examined in a previously published breast cancer containing microarray and patient clinical data set available from the University of North Carolina (UNC), which includes 337 human breast tumours (UNC337) and is available in the Gene Expression Omnibus (GEO) under accession number GEO:( GSE18229 ) [10] . All data sets were median centred within each data set and standardized to zero mean and unit variance before downstream analysis [10] . ANOVA analysis of representative gene expression in tumour samples was determined using the UNC337 gene expression data set. To determine whether the overlap of CtBP target gene lists with other referenced gene lists, is statistically significant in Venn Diagrams, a hypergeometric distribution was calculated to derive the statistical P -value based on 3,7630 TSSs in refseq (HG19, USCS). Analysis of patient survival associated with gene expression from breast cancer data sets was performed using BRB ArrayTools Version: 4.1.0—Beta_3 Release. Affymetrix data sets were downloaded from the NCBI GEO ( http://www.ncbi.nlm.nih.gov/geo/ ). Expression data were loaded into BRB ArrayTools using the Data Import Wizard. U133A probe sets for the individual gene signatures were identified by using the Affymetrix NetAffx Analysis Center Batch Query tool ( http://www.affymetrix.com/analysis/index.affx ). Expression data were filtered to exclude any probe set that was not a component of the signatures tested, and to eliminate any probe set whose expression variation across the data set was P >0.05. Kaplan–Meier analysis was performed using the Survival Risk Prediction tool, specifying two risk groups, with fitting to a Cox proportional hazard model with P -value≤0.05. Distributions of the hazard ratios and the logrank test P -values was determined based on 1,000 Bootstrap samples where each bootstrap sample consists of 50% of cases randomly selected from the whole set [56] . Statistical analysis All the error bars represent the s.d. of the mean from at least three independent biological replicates unless otherwise indicated. Comparison between two groups was done using a two-sided Student’s t test. P -value<0.05 was considered statistically significant. Accession codes: Microarray data have been deposited in the Gene Expression Omnibus database under series accession code GSE36529 . How to cite this article: Di, L-J. et al. Genome-wide profiles of CtBP link metabolism with genome stability and epithelial reprogramming in breast cancer. Nat. Commun. 4:1449 doi: 10.1038/ncomms2438 (2013).